High-quality EuO thin films the easy way via topotactic transformation Epitaxy is widely employed to create highly oriented crystalline films. A less appreciated, but nonetheless powerful means of creating such films is via topotactic transformation, in which a chemical reaction transforms a single crystal of one phase into a single crystal of a different phase, which inherits its orientation from the original crystal. Topotactic reactions may be applied to epitactic films to substitute, add or remove ions to yield epitactic films of different phases. Here we exploit a topotactic reduction reaction to provide a non-ultra-high vacuum (UHV) means of growing highly oriented single crystalline thin films of the easily over-oxidized half-metallic semiconductor europium monoxide (EuO) with a perfection rivalling that of the best films of the same material grown by molecular-beam epitaxy or UHV pulsed-laser deposition. As the technique only requires high-vacuum deposition equipment, it has the potential to drastically improve the accessibility of high-quality single crystalline films of EuO as well as other difficult-to-synthesize compounds. Europium metal can adopt three stable valence states, Eu 2+ in europium monoxide (EuO, rock salt structure, space group Fm m ) (ref. 1 ), Eu 2 2/3+ in Eu 3 O 4 (orthorhombic structure, space group Pnma ) [2] and Eu 3+ in Eu 2 O 3 (monoclinic or cubic structure, space groups C 2/ m or Ia , respectively) [3] , [4] . Of these phases, EuO is scientifically the most interesting compound, mainly because it is a rare example of a high-magnetization ferromagnetic semiconductor (7 μ B per Eu; T C =69 K) (ref. 5 ) which can be epitactically integrated with silicon [6] , GaAs [7] , GaN [6] , graphene [8] , diamond [9] and many oxide substrates. It is a half metal with over 96% spin polarization and can be conductance matched to silicon by rare-earth doping, rendering it an ideal candidate for spintronic applications [6] , [10] . In addition, it shows a plethora of giant transport and magneto-optic properties, which makes it a fascinating material for basic research as well as device applications [6] . As EuO has its highest potential when epitactically integrated with spintronic-relevant semiconductors, the requirements with respect to the structural perfection of EuO films are basically the same as for all other semiconductor applications. Decades of technological innovation make it possible to fabricate silicon and other mainstream semiconductors with unrivalled perfection. For thin films, the standard methods all involve epitaxy—utilizing liquids (liquid-phase epitaxy), gases (vapour-phase epitaxy) or solids (solid-phase epitaxy). In this process, the atoms in the film inherit their crystalline arrangement from the underlying single crystal on which they are deposited and with which they do not react. If the depositing materials react with the substrate, the result is often disastrous to the crystalline perfection of the product formed, but an exception exists: topotaxy. Here the product inherits its highly oriented structure from the single crystal it replaced [11] . Although rare, topotactic transformations can occur as materials oxidize (for example, Fe to FeO, Cu to Cu 2 O) (ref. 12 ), alter their hydrogen content (for example, FeO(OH) to Fe 2 O 3 ) (ref. 11 ), swap anions (for example, ZnS to ZnO) (ref. 13 ) or undergo phase transitions [14] (for example, the α to β transition in quartz) [11] . They are known for many mineral systems (for example, the formation of spinel from sapphire and periclase) [11] , [15] and have even been observed in meteorites [16] . Most involve the substitution or addition of ions to a structure, but examples involving reduction are known [17] , [18] , [19] , [20] , [21] , [22] and have been used to create epitactic films of phases that are otherwise inaccessible including LaNiO 2 , SrFeO 2 , CaFeO 2 and even superlattices of these topotactically transformed phases [23] , [24] , [25] , [26] . This approach is being exploited in thin films due to its experimental simplicity [27] , for example, the formation of SrFeO 3-α F γ from epitactic SrFeO 3- x films, where the corrosive fluorine can be introduced ex situ after the epitactic film growth is complete [28] . In many metal oxides the desired physical properties depend strongly on the structure of the compound, which often can be delicately controlled by altering the oxygen stoichiometry and thereby the oxidation state or valence of the involved metals. Controlling the oxygen stoichiometry is therefore of great importance in the preparation of oxides in the form of epitactic thin films for basic research or applications. For many materials, the desired phase is the fully oxidized one and its synthesis merely requires a sufficiently oxidizing environment during deposition. This makes their growth comparatively easy, for example, by reactive sputtering, molecular-beam epitaxy (MBE) or pulsed-laser deposition (PLD) in a (relatively) high-pressure ambient of oxygen or even ozone. For the case of EuO, however, the phase with the lowest oxidation state shows by far the most interesting physical properties. To access this phase one faces much higher demands, mainly the need to provide a controlled environment that is neither too oxidative nor too reducing during both growth and cooling following growth. In this Article we demonstrate an alternative approach that does not require ultra-high-vacuum (UHV) equipment to grow high-quality EuO films, but can be executed in standard high-vacuum deposition systems, which are much more abundant. This technique allows the growth of single crystalline EuO films by magnetron sputtering under high-vacuum conditions with crystalline quality surpassing that of the best films grown by UHV techniques. The growth mechanism is based on a chemical reduction of an epitactic Eu 2 O 3 precursor film into single crystalline EuO by chemical reduction. As the resulting high-quality EuO film inherits its crystalline structure form the precursor film, the reduction reaction is a topotactic transformation. Stability requirements and growth kinetics At room temperature Eu 2+ is only thermodynamically stable in minuscule oxygen partial pressures (below 10 –64 atm) [29] , making its growth as well as subsequent ex situ processing highly demanding [6] . This instability in ambient conditions has, up to now, limited the growth of epitactic EuO films with high crystalline quality to UHV MBE [6] , [7] , [8] , [9] , [10] , [30] , [31] and UHV PLD [32] , [33] . Sputtering of EuO films from an EuO target [34] , [35] or multiple targets (Eu metal and Eu 2 O 3 ) (refs 36 , 37 ) has been reported, but resulted in polycrystalline, multiphase films, even when grown in a UHV deposition system. For multivalent metals, thermodynamically relevant pressure values can be derived from Ellingham diagrams. According to thermodynamics, at 700 K, europium will only be stable in its lowest oxidation state (Eu 2+ in EuO) if the oxygen partial pressure lies between 5 × 10 –80 and 2 × 10 –57 atm [29] , [38] . For thin-film growth, the kinetics of oxidation are also important [39] , [40] , [41] . To form EuO from incident molecular beams of europium and oxygen, the partial pressure of oxygen must be precisely calibrated so that the ratio of the sticking coefficients of europium atoms and O 2 molecules imping on the film surface per unit time is 2:1. Deviations from this ratio lead to defects such as oxygen vacancies or higher Eu-oxides such as Eu 3 O 4 and Eu 2 O 3 , unless self-limiting processes can be utilized. Because of this difficulty, EuO thin films are typically grown with adsorption-controlled techniques [30] requiring well-controlled oxygen partial pressures in the UHV range and limiting deposition temperatures to values above ∼ 400 °C. Also, epitactic growth of many other multivalent metals requires sophisticated and expensive deposition equipment such as UHV MBE or PLD systems effectively limiting the access to high-quality epitactic films of such materials. Four-circle X-ray diffraction (XRD) structural analysis The crystalline quality of all films was investigated using four-circle XRD. To demonstrate the transformation reaction, two Eu 2 O 3 films were deposited simultaneously on (110) YAlO 3 (ref. 42 ). Sample 1 was then taken out of the sputter system, while (after air exposure) sample 2 was heated back up to T D ≈580 °C and capped with titanium as described in Methods. 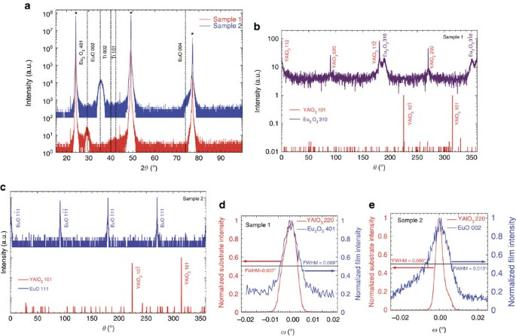Figure 1: Establishing the orientation relationship of the topotactic transformation. (a)θ–2θ-scans of a single-phase (401)-oriented Eu2O3film (sample 1) and a single-phase (001)-oriented EuO film capped with titanium (sample 2) grown on (110) YAlO3. Thickness fringes are present around the EuO 002 peak. Substrate peaks are marked by asterisks. (b)φ-scans of the YAlO3101 and the monoclinic Eu2O3310 families of peaks. These scans demonstrate the epitactic growth of the Eu2O3film with in-plane orientation relationship(scan parameters:;;;). (c)φ-scans of the YAlO3101 and the EuO 111 families of peaks. The four EuO peaks demonstrate the topotactic conversion of Eu2O3into an untwinned (001)-oriented EuO film on the (110) YAlO3substrate with in-plane orientation relationships(scan parameters: 2θEuO=30.08°;ψEuO=52.50°;;). (d) Rocking curves of the YAlO3220 peak and the Eu2O3401 peak, measured on sample 1, respectively. The FWHM of the film peak is comparable to that of the substrate peak, indicating the excellent crystalline quality. (e) Rocking curves of the YAlO3220 peak and the EuO 002 peak, measured on sample 2, respectively. The FWHM of the film peak is only slightly larger than that of the film peak of sample 1. Figure 1a shows the θ –2 θ -scans of both samples. Sample 1 corresponds to (401)-oriented single-phase monoclinic Eu 2 O 3 . The θ –2 θ -scan of sample 2, however, corresponds to a (001)-oriented single-phase EuO film. The orientation relationships between the films and substrates were determined by off-axis XRD scans. Figure 1b shows φ -scans of the YAlO 3 substrate and the Eu 2 O 3 film of sample 1. In combination with calculated orientation relationships ( Supplementary Figs 1 and 2 and Supplementary Table 1 ), the data shows epitactic growth with an in-plane orientation relationship . The φ -scans of sample 2 ( Fig. 1c ) correspond to single crystalline EuO with an in-plane orientation relationship to the substrate of Rocking curves of the Eu 2 O 3 401 peak and the EuO 002 peak ( Fig. 1d,e ) demonstrate the outstanding crystalline quality of the Eu 2 O 3 and the EuO films, respectively. The full width at half maximum (FWHM) of the Eu 2 O 3 401 peak of 0.009° is comparable to that of the substrate (0.007°). The FWHM of 0.013° of the EuO 002 peak of sample 2 is only slightly larger ( Fig. 1e ). For samples where the titanium layer was deposited in situ , directly after the Eu 2 O 3 deposition, a FWHM of the EuO 002 peak as small as 0.004° has been observed using a substrate with a comparably small FWHM. This is the smallest value reported in the literature, smaller even than the best films grown by MBE or UHV PLD [30] , [33] . Using X-ray reflectometry, a root-mean-squared (r.m.s.) interface roughness of 0.28 nm between the EuO film and the TiO x layer was measured. This value is smaller than the r.m.s. roughness of the substrate surface measured by X-ray reflectometry of 0.70 nm, indicating a high-quality interface ( Supplementary Fig. 4 ). Figure 1: Establishing the orientation relationship of the topotactic transformation. ( a ) θ –2 θ -scans of a single-phase (401)-oriented Eu 2 O 3 film (sample 1) and a single-phase (001)-oriented EuO film capped with titanium (sample 2) grown on (110) YAlO 3 . Thickness fringes are present around the EuO 002 peak. Substrate peaks are marked by asterisks. ( b ) φ -scans of the YAlO 3 101 and the monoclinic Eu 2 O 3 310 families of peaks. These scans demonstrate the epitactic growth of the Eu 2 O 3 film with in-plane orientation relationship (scan parameters: ; ; ; ). ( c ) φ -scans of the YAlO 3 101 and the EuO 111 families of peaks. The four EuO peaks demonstrate the topotactic conversion of Eu 2 O 3 into an untwinned (001)-oriented EuO film on the (110) YAlO 3 substrate with in-plane orientation relationships (scan parameters: 2 θ EuO =30.08°; ψ EuO =52.50°; ; ). ( d ) Rocking curves of the YAlO 3 220 peak and the Eu 2 O 3 401 peak, measured on sample 1, respectively. The FWHM of the film peak is comparable to that of the substrate peak, indicating the excellent crystalline quality. ( e ) Rocking curves of the YAlO 3 220 peak and the EuO 002 peak, measured on sample 2, respectively. The FWHM of the film peak is only slightly larger than that of the film peak of sample 1. Full size image As the XRD data demonstrate, it is the hot capping of the Eu 2 O 3 with titanium that leads to a reduction of the precursor films to single crystalline, topotactic, high-quality EuO films. During this reaction the titanium metal is oxidized to TiO x . This reduction induced by the titanium capping is a topotactic transformation, a chemical reaction that results in a material with a crystalline orientation related to the starting product [11] , [43] , [44] . STEM and EELS analysis To verify this transformation mechanism and to characterize the film microstructure, europium valence and interface abruptness, the same samples shown in Fig. 1 were investigated by scanning transmission electron microscopy (STEM) and electron energy-loss spectroscopy (EELS). 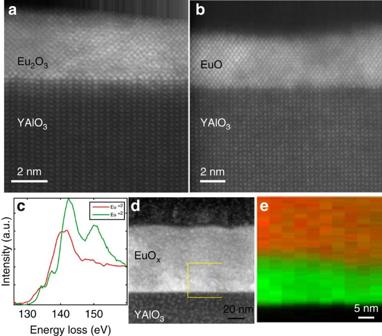Figure 2: Characterization of the europium valence and film microstructure. (a) Cross-sectional HAADF-STEM image of the Eu2O3film (sample 1). (b) Cross-sectional HAADF-STEM image of the transformed EuO film (sample 2) viewed along the [110] zone axis of the EuO film and thezone axis of the YAlO3. SeeSupplementary Fig. 3for a lower magnification STEM image of this same sample showing a larger area. (c) EELS fine structure analysis of the EuO M4.5edge. Distinct EELS fingerprints corresponding to the occurrence of only Eu3+in sample 1 and of only Eu2+in sample 2, respectively. (d) Cross-sectional HAADF-STEM image of a partially reduced EuO film. The EELS analysis was performed on the region indicated by the yellow box. A non-negative nonlinear least squares fit to the components increveals the distribution of the EuO (Eu2+is shown in red) and Eu2O3(Eu3+is shown in green) in the partially reduced film as shown in (e). Streaks at the top of the STEM images are an artifact of post-acquisition drift correction. Figure 2a shows the high-angle annular dark field (HAADF) signal from the Eu 2 O 3 film (sample 1) and Fig. 2b shows the HAADF signal from the EuO film (sample 2). The Eu 2 O 3 film is epitactic to the substrate and exhibits distinct Eu 3+ valence revealed by EELS. The Eu 2+ and Eu 3+ Eu–N 4,5 edges are shown in Fig. 2c [45] , [46] . The transformed EuO film, sample 2, also formed a coherent interface with the YAlO 3 substrate. A diffractogram from the film ( Fig. 1a ) shows a pattern consistent with the EuO rock salt crystal structure. The EELS signal depicted in Fig. 2c shows a distinct fingerprint, consistent with the Eu 2+ state [45] , [46] . Lateral scans across the film did not yield any variations in the europium valence as would be expected for a film with predominately EuO and potentially small remnant inclusions of Eu 2 O 3 (or Eu 3 O 4 ). Therefore, we conclude that the film is phase pure and does not contain any remnant inclusions of Eu 2 O 3 or Eu 3 O 4 within the detection limit of EELS. Figure 2: Characterization of the europium valence and film microstructure. ( a ) Cross-sectional HAADF-STEM image of the Eu 2 O 3 film (sample 1). ( b ) Cross-sectional HAADF-STEM image of the transformed EuO film (sample 2) viewed along the [110] zone axis of the EuO film and the zone axis of the YAlO 3 . See Supplementary Fig. 3 for a lower magnification STEM image of this same sample showing a larger area. ( c ) EELS fine structure analysis of the EuO M 4.5 edge. Distinct EELS fingerprints corresponding to the occurrence of only Eu 3+ in sample 1 and of only Eu 2+ in sample 2, respectively. ( d ) Cross-sectional HAADF-STEM image of a partially reduced EuO film. The EELS analysis was performed on the region indicated by the yellow box. A non-negative nonlinear least squares fit to the components in c reveals the distribution of the EuO (Eu 2+ is shown in red) and Eu 2 O 3 (Eu 3+ is shown in green) in the partially reduced film as shown in ( e ). Streaks at the top of the STEM images are an artifact of post-acquisition drift correction. Full size image The transformation of the Eu 2 O 3 precursor film to EuO is driven by chemical reduction with titanium being the reducing agent. The reduction of Eu 3+ to Eu 2+ is described by the chemical reaction: Eu 2 O 3 +Ti→2 EuO+TiO with ΔG° of −461 and −423 kJ mol −1 at 300 and 900 K, respectively [29] , [38] . The formation of the monoxide of titanium (TiO) is energetically favoured ( Supplementary Table 2 ). From these free energies of reaction and the ideal gas constant R , the equilibrium constant of this reaction can be calculated to be K 300 K =5.9 × 10 80 and K 900 K =1.6 × 10 74 . The equilibrium constant is much larger than one, indicating the almost complete conversion of Eu 3+ into Eu 2+ . Note that the formation of europium metal is thermodynamically disallowed because of the positive value of ΔG° for all corresponding formation reactions ( Supplementary Table 2 ). Presumably the same reason precludes the formation of Eu 3 O 4 , though we are not aware of free energy data for Eu 3 O 4 . As the reduction of Eu 3+ to Eu 2+ requires oxygen diffusion from the precursor film to the titanium capping layer, the transformation propagates from the titanium layer into the Eu 2 O 3 film. Figure 2d shows a HAADF-STEM image and Fig. 2e , the valence analysis of the EELS signal of an only partially reduced film. The EELS signal was fitted with a linear least square optimization to the europium reference spectra shown in Fig. 2c to determine the spatial variance in the europium valence. Close to the titanium layer, only Eu 2+ is present, whereas near the substrate, only Eu 3+ can be found. The depth of the reduction strongly depends on the oxygen diffusion length and hence on the substrate temperature during the titanium deposition. We find that at room temperature <1 nm of the Eu 2 O 3 is reduced to EuO, whereas at 600 °C at least 60 nm of EuO can be transformed. We note that the partially oxidized titanium capping layer protects the EuO film from re-oxidation when exposed to air. This allows ex situ measurements of the films without the need for further protection. Magnetic properties The high crystalline quality results in excellent physical properties of the transformed EuO films. The Curie temperature ( T C ) and the magnetic field dependence of the magnetization ( M ( T ) and M ( μ 0 H )) of the films were determined using superconducting quantum interference device magnetometry. 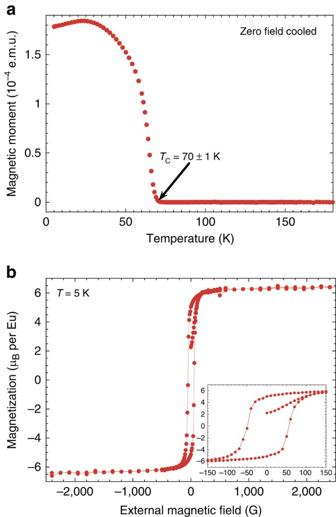Figure 3: Magnetic properties of topotactic EuO. (a) Spontaneous magnetizationM(T) of an EuO film grown on (110) YAlO3via a topotactic transformation, measured using superconducting quantum interference device magnetometry in zero external field. Both the shape of theM(T) curve and the extractedTCis typical of EuO films. The decrease ofM(T) at low temperatures is due to domain effects. (b)M(μ0H) curve of the same sample. The saturation magnetization of the film was determined to beμBper Eu. The inset shows a magnified view of the hysteresis curve, which has a coercive field of 50±10 G. Figure 3a shows a typical zero-field M ( T ) measurement from which T C =70±1 K was determined [47] . This value equals that of bulk EuO (ref. 48 ). Figure 3b shows the in-plane M ( μ 0 H ) characteristic at T =5 K of the same film. The saturation magnetization of μ B per Eu is in good agreement with the expected saturation magnetization of 7 μ B per Eu originating from the 4 f (ref. 7 ) electronic configuration of Eu 2+ (ref. 5 ). The very low coercive field of 50±10 G is again consistent with the excellent crystalline quality of the film. Figure 3: Magnetic properties of topotactic EuO. ( a ) Spontaneous magnetization M ( T ) of an EuO film grown on (110) YAlO 3 via a topotactic transformation, measured using superconducting quantum interference device magnetometry in zero external field. Both the shape of the M ( T ) curve and the extracted T C is typical of EuO films. The decrease of M ( T ) at low temperatures is due to domain effects. ( b ) M ( μ 0 H ) curve of the same sample. The saturation magnetization of the film was determined to be μ B per Eu. The inset shows a magnified view of the hysteresis curve, which has a coercive field of 50±10 G. Full size image From the orientation relationship between the initial epitactic Eu 2 O 3 film and the (110) YAlO 3 substrate on which it was grown (Supplementary Fig. 1) and the orientation relationship of the topotactically transformed EuO film with this same substrate (Supplementary Fig. 2), we know the alignment between the reactant and product phases: with . This orientation relationship is shown in Fig. 4 . Motifs of structural similarity and a reasonable lattice match (–1.0% along and –5.8% along ) are evident between the (401) Eu 2 O 3 and (001) EuO planes. Interestingly, the shortest distance between europium atoms in the Eu 2 O 3 before the topotactic transformation (the direction) ends up being nearly parallel to the shortest distance between europium atoms in the EuO following the transformation (the direction). This same behaviour has also been noted in other topotactic transformations: Fe to FeO (ref. 49 ) and Ba to BaO (ref. 50 ). A plausible pathway for the topotactic transformation between Eu 2 O 3 and EuO is shown in Fig. 4 . The closely packed (401) plane of Eu 2 O 3 in Fig. 4b,c has composition EuO. Shifting the indicated columns of atoms in the (401) plane of Eu 2 O 3 by 1.8 Å along (see Fig. 4c ) results in virtually identical atomic patterns in the (401) Eu 2 O 3 and (001) EuO planes. 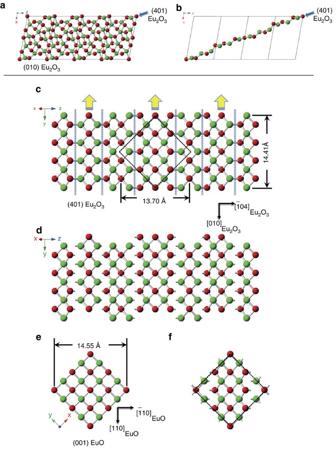Figure 4: A comparison of the atomic arrangements of the (401) Eu2O3and (001) EuO planes. (a) The crystal structure of the monoclinic polymorph of Eu2O3viewed along the [010] zone axis. The unit cell of Eu2O3is outlined with dashed lines and the (401) plane, which is viewed edge-on, is indicated by the blue line. (b) The atoms closest to the chosen (401) plane (the blue line) have overall composition EuO and form a closely packed layer. (c) The (401) plane of atoms selected inbviewed at normal incidence. The atomic arrangement is similar to that of the (001) EuO plane and can be made virtually identical by shifting the columns of atoms between the dashed lines in the direction of the yellow arrows by. (d) The (401) plane of Eu2O3after performing the atomic shifts described inc. (e) The (001) EuO plane. (f) Emphasizes the similarity in atomic arrangement betweendande, by showing the overlap unit cell of shifted. The overlap unit cell betweenand (001)EuOis also shown by the dashed quadrilateral (a rhombus forand a square for (001)EuO) inc, before any shift of the atomic positions. Figure 4: A comparison of the atomic arrangements of the (401) Eu 2 O 3 and (001) EuO planes. ( a ) The crystal structure of the monoclinic polymorph of Eu 2 O 3 viewed along the [010] zone axis. The unit cell of Eu 2 O 3 is outlined with dashed lines and the (401) plane, which is viewed edge-on, is indicated by the blue line. ( b ) The atoms closest to the chosen (401) plane (the blue line) have overall composition EuO and form a closely packed layer. ( c ) The (401) plane of atoms selected in b viewed at normal incidence. The atomic arrangement is similar to that of the (001) EuO plane and can be made virtually identical by shifting the columns of atoms between the dashed lines in the direction of the yellow arrows by . ( d ) The (401) plane of Eu 2 O 3 after performing the atomic shifts described in c . ( e ) The (001) EuO plane. ( f ) Emphasizes the similarity in atomic arrangement between d and e , by showing the overlap unit cell of shifted . The overlap unit cell between and (001) EuO is also shown by the dashed quadrilateral (a rhombus for and a square for (001) EuO ) in c , before any shift of the atomic positions. Full size image In conclusion, we have demonstrated the topotactic transformation of epitactic Eu 2 O 3 films grown on (110) YAlO 3 into high-quality, single crystalline EuO films by a titanium-induced chemical reduction. The approach only requires high-vacuum deposition equipment, overcoming the prior need for UHV deposition systems to grow films of comparable quality. STEM, EELS and superconducting quantum interference device measurements corroborate the growth mechanism and the excellent quality of the transformed EuO films. The method used is general; provided the structures of the precursor and the target films are closely related, the transformations are expected to be topotactic leading to high-quality single crystalline films. Film growth All films were grown in a high-vacuum sputter deposition system (base pressure ≈3 × 10 −7 mbar) using 3′′ targets (99.99% purity). In the course of this study, the sputtering system was equipped with a more powerful vacuum pump, reducing the base pressure to ≈3 × 10 −8 mbar with no detectable changes in film quality. The films were grown on single crystalline YAlO 3 substrates oriented within 0.2° of (110). (110) oriented YAlO 3 provides a rectangular surface net with in-plane lattice constants 7.431 Å along and 7.370 Å along [001] at room temperature [42] . EuO is cubic with lattice constant 5.144 Å at room temperature [1] . The result is a lattice mismatch of 2.1% for and 1.3% for (ref. 6 ). The substrates were glued to a resistive heater using silver paint. The substrate heater was then installed in the deposition system, which was evacuated to its base pressure. The substrates were then heated in vacuum to their deposition temperature ( T D ≈580 °C). During substrate heating the chamber background pressure usually increased to about 5 × 10 −6 mbar. Eu 2 O 3 was deposited for 20 min by reactive radio-frequency magnetron sputtering at a power of P rf =50 W using an Ar/O 2 working gas mixture (total pressure p tot =0.05 mbar). To provide constant growth conditions during the deposition, both working gases were constantly renewed at flow rates of 2.0 sccm. After the Eu 2 O 3 deposition, the films were capped with titanium by d.c. magnetron sputtering (deposition time=4 min, P d.c. =100 W, argon working gas, P tot =0.05 mbar, argon flow=4.0 sccm). Subsequently the heater was switched off and the films were cooled to room temperature in vacuum. How to cite this article: Mairoser, T. et al . High-quality EuO thin films the easy way via topotactic transformation. Nat. Commun. 6:7716 doi: 10.1038/ncomms8716 (2015).